The MHF complex senses branched DNA by binding a pair of crossover DNA duplexes The conserved MHF1–MHF2 (MHF) complex functions in the activation of the Fanconi anaemia pathway of the DNA damage response, in regulating homologous recombination, and in DNA replication fork maintenance. MHF facilitates the processing of multiple types of branched DNAs by the DNA translocase FANCM. Here we report the crystal structure of a human MHF–DNA complex that reveals the DNA-binding mode of MHF. The structure suggests that MHF prefers branched DNA over double-stranded DNA because it engages two duplex arms. Biochemical analyses verify that MHF preferentially engages DNA forks or various four-way junctions independent of the junction-site structure. Furthermore, genetic experiments provide evidence that the observed DNA-binding interface of MHF is important for cellular resistance to DNA damage. These results offer insights into how the MHF complex recognizes branched DNA and stimulates FANCM activity at such a structure to promote genome maintenance. Fanconi anaemia (FA) is a genetic disease characterized by congenital developmental defects, progressive bone marrow failure and early incidence of cancers [1] . Substantial evidence has linked the FA pathway to the repair of DNA interstrand crosslinks [2] . Sixteen FA complementation groups and their corresponding genes have been identified to date [3] , [4] . Several FA proteins (FANCA, -B, -C, -E, -F, -G, -L and -M) and their associated factors form the FA nuclear core complex that mediates the monoubiquitination of the FANCI–FANCD2 (ID) complex, leading to the activation of the FA pathway [5] . FANCM is a crucial member of the FA core complex. Orthologues of FANCM exist in archaebacteria (Hef) and yeast (Mph1 and Fml1) [6] , [7] , [8] , [9] . FANCM and its orthologues possess a DNA-dependent ATPase activity capable of efficiently processing DNA intermediates, for example, the D-loop and Holliday junction (HJ) arising from homologous recombination events, and mediating the reversal of DNA replication fork structures [10] , [11] . These attributes of FANCM and its orthologues are likely to be important for homologous recombination regulation and replication fork repair [9] , [12] . FANCM associates with a pair of histone-fold proteins called MHF1 and MHF2 (refs 13 , 14 ), which form a tetramer harbouring two copies of the heterodimer [15] , [16] . Cells depleted of either MHF protein recapitulate the FANCM sensitivity profile to various DNA-damaging agents and are impaired for FA pathway activation [13] , [14] . The MHF complex (also known as CENP-S and CENP-X) also possesses centromere-specific functions [16] and is responsible for targeting FANCM to these sites [15] . FANCM–MHF has been suggested to facilitate the replication of centromeric DNA. Biochemically, FANCM prefers to bind branched DNA structures such as model HJs and replication forks [11] . The MHF complex also binds DNA and enhances the DNA replication fork reversal and HJ branch migration activities of FANCM [13] , [14] . It has been suggested that MHF confers to FANCM a higher degree of specificity for branched DNAs, which are common intermediates in homologous recombination and replication fork regression [13] , [14] . How the MHF complex differentiates branched DNA from linear DNA is unknown, even though the crystal structures of MHF from different species [15] , [16] , [17] have shown a tetrameric histone-fold arrangement with a potential DNA-binding patch. To understand the mechanism by which MHF senses branched DNA, we used a combination of X-ray crystallographic, biochemical, single-molecule and in vivo functional studies to investigate the interaction between human MHF and various forms of DNA. Our results support a model wherein MHF recognizes a pair of DNA duplex arms to stimulate FANCM activity at branched DNA. Crystal structures of apo-MHF and its complex with DNA To illuminate the MHF–DNA interaction, we determined the structures of human MHF in three crystal forms and a 26-bp double-stranded DNA (dsDNA)–MHF complex in two crystal forms ( Fig. 1a , Supplementary Fig. 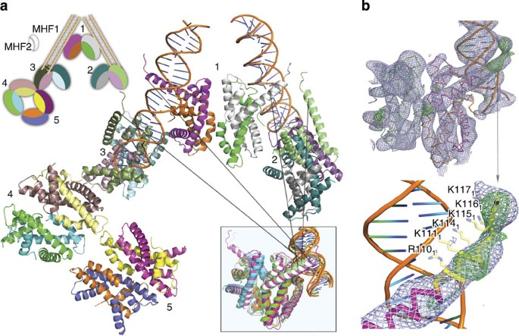Figure 1: Crystal structure of the MHF–DNA complex. (a) The overall structure in the asymmetric unit of the MHF–DNA1 crystal. Two DNA duplexes (brown) and five MHF tetramers (labelled 1–5) are shown in ribbon representation. The top left inset shows the schematic view of the MHF complex (black and white ovals) and the organization of the components of the MHF–DNA complex (coloured). The bottom right inset shows the superposition of the four observed MHF–DNA interaction interfaces. MHF tetramers 1 (two sites), 2 and 3 with associated DNAs are used in this comparison and the arrows point to their positions in the MHF–DNA complex. (b) Unbiased electron density of the MHF–DNA interaction site. Simulated annealing omit map (blue mesh, 2mFo-DFc contoured at 1.1σ, 5 Å around the molecules) was calculated with the displayed MHF tetramer 3 (wire representation) and DNA region (ribbon representation) omitted in the MHF–DNA2 structure. mFo-DFc difference density (green mesh, 2.6σ, 5 Å around the molecules) was generated before any of the C terminus (yellow) was built. Top panel, the overall MHF tetramer–DNA interaction site. Bottom panel, a close-up view of the unbiased electron density around the MHF1 C-terminal region (4 Å around MHF1). The side chains of the positively charged residues (semitransparent sticks) are shown in preferred rotamer positions. S1 and Table 1 ). The MHF apo-structures diffracted to resolutions of 2.5–1.8 Å, with tetrameric MHF structures nearly identical to previously published apo-MHF structures (Cα root mean square deviation: 0.5–1.1 Å) [15] , [16] , [17] . The two MHF–DNA complex crystals, named MHF–DNA1 and MHF–DNA2, diffracted to resolutions of 7.2 and 6.5 Å, respectively. MHF–DNA2 is related to MHF–DNA1 by doubling the unit cell dimension in the c axis due to a translational non-crystallographic symmetry (NCS). Apart from this translational doubling of the unit cell content, the molecules in the two crystals have virtually identical conformations and packing environment. For clarity, we use MHF–DNA1 to describe the structure. The asymmetric unit of the crystal contains two DNA duplexes and five MHF tetramers (labelled 1–5) in three interaction scenarios: MHF tetramer 1 contacts two DNA duplexes, one on each side of the tetramer (double-side binding); each of the MHF tetramers 2 and 3 interacts with one DNA duplex on one side of the tetramer (single-side binding); the MHF tetramers 4 and 5 do not interact with DNA. The excess MHF molecules in the crystal are likely to be due to the length of the dsDNA allowing for the binding of multiple MHFs and also due to crystal packing. Figure 1: Crystal structure of the MHF–DNA complex. ( a ) The overall structure in the asymmetric unit of the MHF–DNA1 crystal. Two DNA duplexes (brown) and five MHF tetramers (labelled 1–5) are shown in ribbon representation. The top left inset shows the schematic view of the MHF complex (black and white ovals) and the organization of the components of the MHF–DNA complex (coloured). The bottom right inset shows the superposition of the four observed MHF–DNA interaction interfaces. MHF tetramers 1 (two sites), 2 and 3 with associated DNAs are used in this comparison and the arrows point to their positions in the MHF–DNA complex. ( b ) Unbiased electron density of the MHF–DNA interaction site. Simulated annealing omit map (blue mesh, 2mFo-DFc contoured at 1.1 σ , 5 Å around the molecules) was calculated with the displayed MHF tetramer 3 (wire representation) and DNA region (ribbon representation) omitted in the MHF–DNA2 structure. mFo-DFc difference density (green mesh, 2.6 σ , 5 Å around the molecules) was generated before any of the C terminus (yellow) was built. Top panel, the overall MHF tetramer–DNA interaction site. Bottom panel, a close-up view of the unbiased electron density around the MHF1 C-terminal region (4 Å around MHF1). The side chains of the positively charged residues (semitransparent sticks) are shown in preferred rotamer positions. Full size image Table 1 Data collection and refinement statistics. Full size table The MHF–DNA complex structure has a very defined conformation with excellent electron density, in which the secondary structural elements of MHF and DNA major/minor grooves are clearly discernable ( Fig. 1b and Supplementary Fig. S2 ). Although side-chain information cannot be directly revealed at 6.5–7 Å resolution, the well-defined secondary structure elements allow for accurate estimate of the side-chain locations using the apo-MHF structures as reference. The MHF tetramers in the DNA complex crystal adopt similar conformations to the published apo-MHF structures ( Supplementary Fig. S1d ), with slight structural variations (Cα root mean square deviation: 2.1–2.7 Å) possibly due to DNA-binding perturbations and/or intrinsic positional uncertainties at 6.5–7 Å resolution. It is likely to be that there are local differences at the DNA-binding interface of MHF with or without bound DNA; however, at our resolution we cannot resolve such detailed differences. The quality and correctness of the structure determination are demonstrated by the unambiguous simulated annealing omit map ( Fig. 1b and Supplementary Fig. S2 ), unbiased electron density for DNA at positions without models ( Supplementary Fig. S2 ), as well as good refinement statistics ( R / R free of 26.8/28.8% for MHF–DNA1, Table 1 ). In addition, unbiased difference electron density for residues 107–118 in the previously unobserved carboxy terminus of MHF1 is clearly visible without any prior model information ( Fig. 1b ; discussed below), further validating the structure. The DNA-binding interface on MHF A conserved MHF–DNA interaction is observed for both the single- and double-sided binding scenarios in the crystals. A superposition of all the independent MHF–DNA interfaces clearly reveals the conserved DNA-binding mode of MHF ( Fig. 1a inset). The MHF–DNA interface buries 1,040 Å 2 surface area per interaction site. To simplify the description, we divide the positively charged circumference of the MHF tetramer into top (K73, R74, K94, K99 and R110 of MHF1), shoulder (R18 of MHF1 and R17, R11, K12, K27, K29 and H20 of MHF2), arm (MHF1 C terminus) and bottom (K44 of MHF1 and R64 of MHF2) patches ( Fig. 2a ). The MHF residues at the DNA-binding interface are conserved among many vertebrates, including human, chimpanzee, mouse, bird and fish ( Supplementary Fig. S3a,b ). 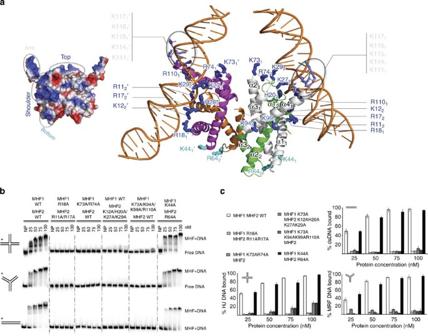Figure 2: The positively charged patches of MHF are essential for DNA binding. Overall (top left inset, shown as electrostatic surface; blue: positive, red: negative) and detailed (ribbon representation) views of the MHF–DNA interface (tetramer 1 in MHF–DNA1). (a) The critical top and shoulder residues (stick representation) for DNA binding are in blue, the positively charged arm (highlighted by ovals) residues are in light-blue sticks and those residues that do not affect DNA binding are in cyan. (b) Electrophoretic mobility shift analysis of MHF mutants with various DNA substrates (the schematics of the HJ DNA, Y-DNA and dsDNA are shown on the left with the radiolabelled terminus indicated by an asterisk). The substrates (30 nM) were incubated with increasing amounts of WT or mutant-MHF (25, 50, 75 and 100 nM) and analysed. NP, no protein added. (c) The results were quantified and plotted in the bar graphs. Error bars were generated from the s.d. in triplicate experiments. Figure 2: The positively charged patches of MHF are essential for DNA binding. Overall (top left inset, shown as electrostatic surface; blue: positive, red: negative) and detailed (ribbon representation) views of the MHF–DNA interface (tetramer 1 in MHF–DNA1). ( a ) The critical top and shoulder residues (stick representation) for DNA binding are in blue, the positively charged arm (highlighted by ovals) residues are in light-blue sticks and those residues that do not affect DNA binding are in cyan. ( b ) Electrophoretic mobility shift analysis of MHF mutants with various DNA substrates (the schematics of the HJ DNA, Y-DNA and dsDNA are shown on the left with the radiolabelled terminus indicated by an asterisk). The substrates (30 nM) were incubated with increasing amounts of WT or mutant-MHF (25, 50, 75 and 100 nM) and analysed. NP, no protein added. ( c ) The results were quantified and plotted in the bar graphs. Error bars were generated from the s.d. in triplicate experiments. Full size image The MHF–DNA structure shows that residues in the top, shoulder and arm patches of MHF are close to the DNA backbone, whereas the bottom patch is situated away from the binding interface ( Fig. 2a ). Although the MHF–DNA interface covers both the minor and the major grooves of DNA, MHF primarily interacts with DNA sugar-phosphate backbones and there does not appear to be base-specific interactions in the grooves. This backbone-only recognition is a common feature of nonspecific DNA-binding proteins. To validate the structural observation, we systematically investigated the charged MHF residues involved in DNA binding ( Fig. 2b,c ). As predicted from the structure, mutations of the residues in the shoulder and top patches abolish MHF binding to HJ, forked and duplex DNAs [14] , whereas mutations in the bottom patch have little effect on DNA binding ( Fig. 2b,c ). The positively charged C-terminal region of MHF1, which is disordered in all apo-MHF structures, also engages in interactions with DNA and becomes structured. Extending from the end of the structured apo-MHF1 C-terminal α-helix, residues 107–118 form ~2 more α-helical turns followed by a loop region. These newly structured residues are located next to the negative-charged DNA phosphate backbone ( Fig. 1b ). Although we cannot accurately model side chains at the low resolution, it is evident that the positive-charged clusters (including R110, K111, K114, K115, K116 and K117 of MHF1) in this arm region are positioned close to the DNA backbone, forming potential electrostatic interactions ( Fig. 1b ). The MHF1 C terminus is only observed at the sites where the molecule interacts with DNA, whereas it remains disordered in those MHF1 copies in the crystal that do not contact DNA. This is consistent with and provides a structural explanation for the observation that the C-terminal region of MHF1 is necessary for DNA binding [13] . DNA condensation by binding to both sides of MHF In the crystal structure, MHF tetramer 1 ( Fig. 1a ) engages a pair of DNA duplexes through the positively charged patches on the side and upper circumference of the MHF tetramer, as well as the MHF1 C-terminal arm ( Figs 2a and 3a ). Interestingly, the two DNA helices are not coplanar but are oriented in a stacked conformation with the helical paths of the duplexes closely packing against each other ( Fig. 3a ). A potential consequence of DNA binding by both sides of the MHF tetramer is the condensation of long DNA through bending and looping. Indeed, dsDNA condensing by MHF has been observed by electron microscopy [14] . 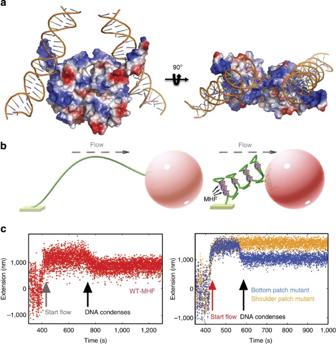Figure 3: MHF condenses dsDNA. (a) Front and top views of the electrostatic interaction between the MHF tetramer (tetramer 1 from MHF–DNA1, surface representation, blue: positive charge, red: negative) and two DNA duplexes. (b,c) Single-molecule TPFS assay of the effect of MHF binding on long dsDNA chains. (b) Schematic of the TPFS assay of DNA condensation by MHF: the optical beads are shown as pink spheres, the DNA is shown as green strings, MHF tetramers are shown in surface representation, the applied flow is shown in grey arrows. The flow force was calibrated inSupplementary Fig. S4. (c) The dsDNA ligand (4,200 bp) was subjected to a fluid flow containing either WT (red), the shoulder patch mutant (R18A/R11A/R17A, blue) or the bottom-patch mutant (K44A/R64A, brown) of MHF. The WT and the bottom-patch mutant of MHF capable of binding DNA cause a significant shortening of the DNA chain, whereas the shoulder patch mutant deficient in DNA binding does not. Figure 3: MHF condenses dsDNA. ( a ) Front and top views of the electrostatic interaction between the MHF tetramer (tetramer 1 from MHF–DNA1, surface representation, blue: positive charge, red: negative) and two DNA duplexes. ( b , c ) Single-molecule TPFS assay of the effect of MHF binding on long dsDNA chains. ( b ) Schematic of the TPFS assay of DNA condensation by MHF: the optical beads are shown as pink spheres, the DNA is shown as green strings, MHF tetramers are shown in surface representation, the applied flow is shown in grey arrows. The flow force was calibrated in Supplementary Fig. S4 . ( c ) The dsDNA ligand (4,200 bp) was subjected to a fluid flow containing either WT (red), the shoulder patch mutant (R18A/R11A/R17A, blue) or the bottom-patch mutant (K44A/R64A, brown) of MHF. The WT and the bottom-patch mutant of MHF capable of binding DNA cause a significant shortening of the DNA chain, whereas the shoulder patch mutant deficient in DNA binding does not. Full size image We conducted single-molecule experiments to further verify the condensation of DNA by MHF. We used the single-molecule technique of tethered particle-flow stretching (TPFS) [19] to show that MHF association indeed induces the shortening of dsDNA ( Fig. 3b,c ). In the TPFS experiment, one end of a dsDNA (4,200 bp) was fixed and the other end was tethered to an optically visible bead, whose position was recorded throughout the experiment. The flexible DNA was stretched to an extended conformation by a calibrated constant flow force of ~0.5 pN ( Supplementary Fig. S4 ). The introduction of MHF led to a significant contraction of the DNA chain by approximately a third of its length (~1,400 bps) in our experimental setup ( Fig. 3c ). The DNA condensation was indeed caused by MHF binding, as revealed by testing MHF mutants ( Fig. 3c ). Specifically, a shoulder patch mutant of MHF (R18A of MHF1 and R11A/R17A of MHF2) deficient in DNA binding failed to condense the DNA, whereas a bottom-patch mutant that retains DNA binding (K44A of MHF1 and R64A of MHF2) was proficient in this regard ( Fig. 3c ). MHF and MHF–FANCM complexes prefer branched DNA over dsDNA The architecture of the MHF–DNA interaction ( Fig. 2a ) strongly suggests an ability of MHF to specifically engage branched DNAs [14] , as both sides of MHF are available for simultaneous DNA binding. To assess the relative affinity of the MHF complex for branched versus linear dsDNA, we performed electrophoretic mobility shift assays with MHF and three different substrates: dsDNA, DNA fork and HJ ( Fig. 4a,b ). The results revealed the order of MHF-binding preference as HJ>DNA fork>dsDNA. We then performed competition assays in which a nucleoprotein complex of MHF with radiolabelled dsDNA was challenged with either cold dsDNA or HJ ( Fig. 4c ). The results clearly showed that HJ is a much better competitor than dsDNA ( Fig. 4d ). At 30 nM cold competitor concentration, which was the same as that of the radiolabelled dsDNA, there was an ~5-fold increase in the amount of released radiolabelled DNA when challenged with HJ versus dsDNA ( Fig. 4d ). 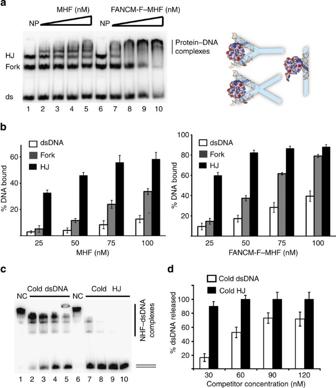Figure 4: MHF binds branched DNA preferentially over dsDNA. (a) Left, analysis of MHF and FANCM-F/MHF complex for binding dsDNA, forked DNA and HJ DNA. Radiolabelled DNA substrates (30 nM each) were incubated with increasing amounts of MHF (lanes 2–5) or FANCM-F/MHF complex (lanes 7–10) in the presence of 150 mM KCl. NP, no protein added (lanes 1 and 6). Right, schematic depicting binding of MHF to forked DNA, HJ or dsDNA; the charged surface is generated from MHF–DNA1. MHF tetramers are shown as electrostatic surfaces, the observed DNA duplexes are shown as brown helices and the DNA substrates used in mobility shift assays are illustrated as cyan bars. (b) Quantification of the results is shown in the bar graphs. Error bars were generated from the s.d. in triplicate experiments. The left panel shows the data for MHF alone, whereas the right panel shows the data for the FANCM-F/MHF complex. (c) Experiments in which a preformed MHF–dsDNA nucleoprotein complex was challenged with a cold DNA substrate. MHF complex (100 nM) was preincubated with radiolabelled dsDNA (30 nM). Increasing amounts of unlabelled dsDNA (lanes 2–5) or HJ (lanes 7–10) were added (30, 60, 90 and 120 nM). NC, control with no DNA competitor. (d) Quantification of the results shown inc. Error bars were generated from the s.d. in triplicate experiments. Figure 4: MHF binds branched DNA preferentially over dsDNA. ( a ) Left, analysis of MHF and FANCM-F/MHF complex for binding dsDNA, forked DNA and HJ DNA. Radiolabelled DNA substrates (30 nM each) were incubated with increasing amounts of MHF (lanes 2–5) or FANCM-F/MHF complex (lanes 7–10) in the presence of 150 mM KCl. NP, no protein added (lanes 1 and 6). Right, schematic depicting binding of MHF to forked DNA, HJ or dsDNA; the charged surface is generated from MHF–DNA1. MHF tetramers are shown as electrostatic surfaces, the observed DNA duplexes are shown as brown helices and the DNA substrates used in mobility shift assays are illustrated as cyan bars. ( b ) Quantification of the results is shown in the bar graphs. Error bars were generated from the s.d. in triplicate experiments. The left panel shows the data for MHF alone, whereas the right panel shows the data for the FANCM-F/MHF complex. ( c ) Experiments in which a preformed MHF–dsDNA nucleoprotein complex was challenged with a cold DNA substrate. MHF complex (100 nM) was preincubated with radiolabelled dsDNA (30 nM). Increasing amounts of unlabelled dsDNA (lanes 2–5) or HJ (lanes 7–10) were added (30, 60, 90 and 120 nM). NC, control with no DNA competitor. ( d ) Quantification of the results shown in c . Error bars were generated from the s.d. in triplicate experiments. Full size image As MHF interacts with FANCM and stimulates its DNA branch migration activity [13] , [14] , we investigated whether the presence of MHF-interacting FANCM fragment (FANCM-F) changes the DNA-binding properties of MHF. We performed the same competition experiments with the complex of MHF and the FANCM fragment (spanning residues 661–800) that harbours the MHF1 interaction domain [14] . Although this fragment of FANCM does not bind DNA on its own ( Supplementary Fig. S5a ), the FANCM-F/MHF complex, when compared with MHF alone, has an enhanced DNA-binding ability ( Fig. 4a,b and Supplementary Fig. S5b ). FANCM-F/MHF shows the same DNA-binding preference as MHF, that is, HJ>DNA fork>dsDNA ( Fig. 4a,b ). MHF preference to branched DNA with adjacent duplexes We notice that the MHF tetramer 1 orients the pair of bound DNA duplexes at a ~55° angle ( Fig. 5a ), which resembles the angle between the two arms of the four-way junction DNA, three-way DNA junction and paused DNA fork in the ‘stacked X’ conformation previously observed in crystal structures [20] , [21] , [22] . The observed angle is also close to the angle of ~60° of the HJ and three-way junction in solution [23] , [24] . This broad geometry resemblance may explain the preference of MHF for branched DNA substrates, where two adjacent duplexes on one side of the junction are bound simultaneously by one MHF tetramer. This would provide a general mechanism by which MHF engages a pair of crossover duplexes in branched DNA structures regardless of the overall architecture of the DNA. 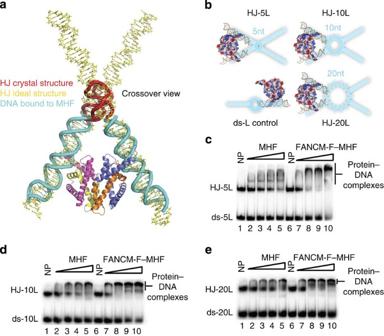Figure 5: MHF specifically engages two arms of a DNA junction. (a) The geometry resemblance between the MHF-bound DNA duplex pair (cyan helices) and the two arms of an ideal HJ DNA (yellow sticks) generated based on the HJ crystal structure (red helices; PDB ID: 3IGT). The DNA-bound MHF tetramer 1 from MHF–DNA1 is shown. (b) Schematic representation of the substrates used. MHF tetramers are shown as electrostatic surfaces, the observed DNA duplexes are shown as brown cartoons and the DNA substrates are illustrated in cyan with the duplex regions as straight bars and the central bubble regions as jagged lines. Analyses of MHF and FANCM-F/MHF for binding the ds-5L and HJ-5L substrates (c), the ds-10L and HJ-10L substrates (d), and the ds-20L and HJ-20L substrates (e). The radiolabelled DNA substrates (30 nM each) were incubated with increasing amounts of MHF (lanes 2–5) or FANCM-F/MHF complex (lanes 7–10) in the presence of 150 mM KCl. NP, no protein added (lanes 1 and 6). Quantification of the results is shown inSupplementary Fig. S4. Figure 5: MHF specifically engages two arms of a DNA junction. ( a ) The geometry resemblance between the MHF-bound DNA duplex pair (cyan helices) and the two arms of an ideal HJ DNA (yellow sticks) generated based on the HJ crystal structure (red helices; PDB ID: 3IGT). The DNA-bound MHF tetramer 1 from MHF–DNA1 is shown. ( b ) Schematic representation of the substrates used. MHF tetramers are shown as electrostatic surfaces, the observed DNA duplexes are shown as brown cartoons and the DNA substrates are illustrated in cyan with the duplex regions as straight bars and the central bubble regions as jagged lines. Analyses of MHF and FANCM-F/MHF for binding the ds-5L and HJ-5L substrates ( c ), the ds-10L and HJ-10L substrates ( d ), and the ds-20L and HJ-20L substrates ( e ). The radiolabelled DNA substrates (30 nM each) were incubated with increasing amounts of MHF (lanes 2–5) or FANCM-F/MHF complex (lanes 7–10) in the presence of 150 mM KCl. NP, no protein added (lanes 1 and 6). Quantification of the results is shown in Supplementary Fig. S4 . Full size image To verify that engagement of duplex arms by MHF is independent of the architecture of the junction point, we assembled HJ-like substrates with a 5-, 10- or 20-nucleotide-long unpaired bubble region at the junction site ( Fig. 5b ). Electrophoretic mobility shift assay experiments with these HJ-like substrates and control linear duplexes with the same size of DNA bubble revealed that the branched HJ-like DNA remains the preferred substrate in each case ( Fig. 5c–e and Supplementary Fig. S6 ). As observed before ( Fig. 4a,b ), the presence of FANCM-F fragment increases DNA-binding affinity but does not change substrate preference ( Fig. 5c–e and Supplementary Fig. S6 ). These data provide additional support to the premise that the preference of MHF and MHF–FANCM for branched DNA structures stems from their ability to simultaneously engage two crossed duplex arms. The MHF–DNA-binding interface is functionally important It has been reported that the interaction of MHF with FANCM is important for the upregulation of the DNA branch migration activity of FANCM [13] , [14] . To test the importance of the observed MHF–DNA interaction in FANCM stimulation, we performed branch migration assays with FANCM alone or together with either wild type (WT) or various mutants of MHF. We used in these reactions a radiolabelled model movable replication fork (MRF) as the substrate [11] , [13] . Although MHF enhanced the branch migration activity of FANCM, the top and shoulder patch mutants that are deficient in DNA binding (R18A/R11A/R17A, K73A/K94A/K99A/R110A, K73A/R74A and K12A/H20A/K27A/K29A) failed to do so. Consistently, the bottom-patch MHF mutant that is DNA-binding proficient (K44A/R64A) stimulated FANCM normally ( Fig. 6a–d ). Importantly, all the mutants preserve the WT oligomerization state ( Supplementary Fig. S3c ) and interact with FANCM as well as WT MHF ( Fig. 6e–h ), suggesting the overall structure is not significantly perturbed by any of these mutations. These results demonstrate that the FANCM stimulatory effect of MHF requires its DNA-binding activity. 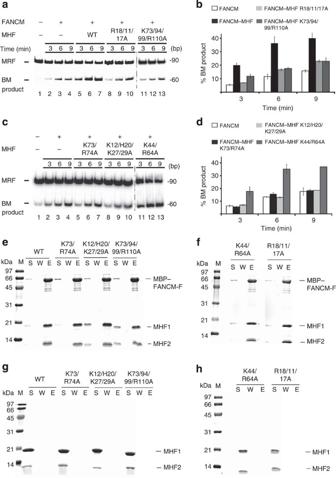Figure 6: DNA binding by MHF enhances FANCM-mediated DNA branch migration but does not correlate with FANCM binding. (a) FANCM (lanes 2–4) or FANCM with either WT MHF (lanes 5–7) or MHF mutants (R18/11A/17A, lanes 8–10 and K73/94/99/R110A, lanes 11–13) was tested for branch migration (BM) activity as a function of time. The concentration of FANCM and MHF (WT or mutant) was 10 nM and of MRF was 5 nM. ATP was present in all the reactions. (c) BM reactions were conducted with FANCM (lanes 2–4) or with FANCM and MHF mutants (K73/R74A, lanes 5–7; K12/H20/K27/29A, lanes 8–10; and K44/R64A, lanes 11–13) as ina. (b,d) Quantification of the data shown inaandc, respectively. Error bars were generated from the s.d. in triplicate experiments. (e–h) Pull-down assays showing that the MHF mutants retain FANCM-binding activity. (e,f) Ten micrograms of WT MHF or MHF mutant as labelled was incubated with the same molar ratio of MBP-His-FANCM-F (FANCM fragments 661–800) before it was bound to amylose agarose resin (10 μl; New England Biolabs). 15% of the supernatant (S) and elution (E) fractions, and 2% of total wash (W) fraction were analysed by SDS–PAGE followed by Coomassie blue staining. (g,h) Control experiments showing that the MHF mutants were not retained on the amylose resin without the inclusion of the MBP-tagged FANCM-F. Figure 6: DNA binding by MHF enhances FANCM-mediated DNA branch migration but does not correlate with FANCM binding. ( a ) FANCM (lanes 2–4) or FANCM with either WT MHF (lanes 5–7) or MHF mutants (R18/11A/17A, lanes 8–10 and K73/94/99/R110A, lanes 11–13) was tested for branch migration (BM) activity as a function of time. The concentration of FANCM and MHF (WT or mutant) was 10 nM and of MRF was 5 nM. ATP was present in all the reactions. ( c ) BM reactions were conducted with FANCM (lanes 2–4) or with FANCM and MHF mutants (K73/R74A, lanes 5–7; K12/H20/K27/29A, lanes 8–10; and K44/R64A, lanes 11–13) as in a . ( b , d ) Quantification of the data shown in a and c , respectively. Error bars were generated from the s.d. in triplicate experiments. ( e – h ) Pull-down assays showing that the MHF mutants retain FANCM-binding activity. ( e , f ) Ten micrograms of WT MHF or MHF mutant as labelled was incubated with the same molar ratio of MBP-His-FANCM-F (FANCM fragments 661–800) before it was bound to amylose agarose resin (10 μl; New England Biolabs). 15% of the supernatant (S) and elution (E) fractions, and 2% of total wash (W) fraction were analysed by SDS–PAGE followed by Coomassie blue staining. ( g , h ) Control experiments showing that the MHF mutants were not retained on the amylose resin without the inclusion of the MBP-tagged FANCM-F. Full size image We also validated the biological relevance of the MHF–DNA-binding attribute using cell-based assays. For this, we depleted MHF1 endogenous to HeLa cells via short hairpin RNA (shRNA) treatment ( Supplementary Fig. S7a ) and then examined the ability of ectopically expressed, shRNA-resistant WT or mutant-MHF1 to complement the phenotypes stemming from MHF1 ablation. By co-immunoprecipitation, we verified that the DNA-binding-deficient mutant (K73A/K94A/K99A/R110A of MHF1) is incorporated into the higher-order complex with MHF2, FANCM and FAAP24 ( Fig. 7a ). However, cells expressing the mutant protein remained sensitive to camptothecin and mitomycin C (MMC; Fig. 7c ). Consistent with these results, the mutant MHF1 failed to support FANCD2 monoubiquitination ( Fig. 7b ) and was also defective for chromatin co-localization of FA core complex members ( Fig. 7d ) on MMC treatment. We note that previous work [13] , [14] , [15] also showed that mutations in the top patch residues (K73 and R74 of MHF1) render the MHF complex impaired in DNA binding, chromatin co-localization of FA proteins and FANCD2 monoubiquitination at cellular level. Therefore, the DNA-binding interface observed in the MHF complex is clearly important for the functional integrity of the FA pathway of DNA repair. 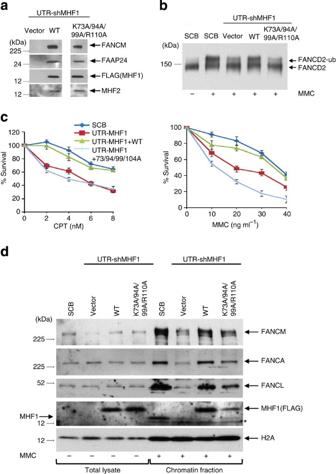Figure 7: Cellular phenotypes of MHF–DNA-binding mutants. (a) The MHF1 DNA-binding mutant (K73A/K94A/K99A/R110A) is proficient in interactions with MHF2 and FANCM-FAAP24. HeLa cells transduced with lentiviruses carrying MHF1-UTR were further transduced with retroviruses carrying empty vector (lane 1), Flag-WT-MHF1 (lane 2) or Flag-MHF1 mutant (lane 3), and the anti-Flag-immunoprecipitated protein complex was analysed by immunoblotting with the indicated antibodies. (b) The MHF1 DNA-binding mutation (K73A/K94A/K99A/R110A) affects FANCD2 monoubiquitination. Immunoblottting showing impaired FANCD2 monoubiquitination in the MHF1 mutant. HeLa cells were transduced with lentiviruses carrying either control shRNA (SCB, lanes 1–2) or MHF1-UTR (UTR-shMHF1, lanes 3–5). Next, Hela-MHF1-UTR cells were transduced with retroviruses carrying either empty vector (vector, lane 3), shRNA-resistant WT-MHF1 cDNA (WT, lane 4) or mutant-MHF (K73A/K94A/K99A/R110A, lane 5). Cells were treated with 100 ng ml−1MMC for 16 h and blotted by anti-FANCD2 antibody. FANCD2-ub, monoubiquitinated FANCD2. (c) DNA binding by MHF is required for cellular resistance to DNA-damaging agents. HeLa cells with endogenous MHF1 depleted by shRNA treatment and expressing either WT or the DNA-binding mutant of MHF1 (seebfor details) were treated with the indicated concentration of camptothecin (CPT) or MMC. Visible colonies from 200 cells were counted after 10 days. The data represent the per cent survival, as compared with untreated cells. Each experiment was performed in triplicate and mean values are shown with s.d. (d) Immunoblotting showing the levels of FA core complex members in total lysate and chromatin fraction. HeLa cells were transduced with lentiviruses carrying either control shRNA (SCB) or MHF1-UTR (UTR-shMHF1). Next, Hela-MHF1-UTR cells were transduced with retroviruses carrying empty vector (vector), shRNA-resistant WT-MHF1 cDNA (WT) or mutant-MHF (K73A/K94A/K99A/R110A). Cells were treated with 100 ng ml−1MMC for 16 h, followed by cellular fractionation into total lysate and chromatin fraction. The relevant proteins were revealed by immunoblotting. H2A serves as loading control and a marker for the chromatin fraction. *A nonspecific crossreactive band. Figure 7: Cellular phenotypes of MHF–DNA-binding mutants. ( a ) The MHF1 DNA-binding mutant (K73A/K94A/K99A/R110A) is proficient in interactions with MHF2 and FANCM-FAAP24. HeLa cells transduced with lentiviruses carrying MHF1-UTR were further transduced with retroviruses carrying empty vector (lane 1), Flag-WT-MHF1 (lane 2) or Flag-MHF1 mutant (lane 3), and the anti-Flag-immunoprecipitated protein complex was analysed by immunoblotting with the indicated antibodies. ( b ) The MHF1 DNA-binding mutation (K73A/K94A/K99A/R110A) affects FANCD2 monoubiquitination. Immunoblottting showing impaired FANCD2 monoubiquitination in the MHF1 mutant. HeLa cells were transduced with lentiviruses carrying either control shRNA (SCB, lanes 1–2) or MHF1-UTR (UTR-shMHF1, lanes 3–5). Next, Hela-MHF1-UTR cells were transduced with retroviruses carrying either empty vector (vector, lane 3), shRNA-resistant WT-MHF1 cDNA (WT, lane 4) or mutant-MHF (K73A/K94A/K99A/R110A, lane 5). Cells were treated with 100 ng ml −1 MMC for 16 h and blotted by anti-FANCD2 antibody. FANCD2-ub, monoubiquitinated FANCD2. ( c ) DNA binding by MHF is required for cellular resistance to DNA-damaging agents. HeLa cells with endogenous MHF1 depleted by shRNA treatment and expressing either WT or the DNA-binding mutant of MHF1 (see b for details) were treated with the indicated concentration of camptothecin (CPT) or MMC. Visible colonies from 200 cells were counted after 10 days. The data represent the per cent survival, as compared with untreated cells. Each experiment was performed in triplicate and mean values are shown with s.d. ( d ) Immunoblotting showing the levels of FA core complex members in total lysate and chromatin fraction. HeLa cells were transduced with lentiviruses carrying either control shRNA (SCB) or MHF1-UTR (UTR-shMHF1). Next, Hela-MHF1-UTR cells were transduced with retroviruses carrying empty vector (vector), shRNA-resistant WT-MHF1 cDNA (WT) or mutant-MHF (K73A/K94A/K99A/R110A). Cells were treated with 100 ng ml −1 MMC for 16 h, followed by cellular fractionation into total lysate and chromatin fraction. The relevant proteins were revealed by immunoblotting. H2A serves as loading control and a marker for the chromatin fraction. *A nonspecific crossreactive band. Full size image MHF plays an important role in facilitating the processing of multiple types of branched DNAs in the FA pathway of DNA damage repair. Our X-ray crystallographic studies on human MHF provide evidence that MHF recognizes two crossover DNA duplexes, a common feature in various DNA junction structures that occur during DNA replication and repair in cells. This attribute of MHF would enable MHF to recognize a wide range of branched DNA junction structures of different architectures, such as forked and HJ DNAs. The preference of MHF for branched DNA suggests a potential mechanism by which this protein complex facilitates the localization of FANCM to DNA junctions. We have analysed possible protein–DNA interactions at a DNA junction using structural information from our MHF–DNA complex, the MHF–FANCM complex [15] , an ideal HJ DNA, and a homology-modelled FANCM helicase domain based on the crystal structure of Hef [25] ( Fig. 8a ). According to our model, simultaneous interactions of MHF with two DNA arms and FANCM promote the recruitment of FANCM to the DNA junction ( Fig. 8a,b ). The MHF–FANCM interaction could further help position the helicase domain of FANCM at the junction crossover point to mediate DNA branch migration, as the distance between the MHF-binding site and the DNA junction appears to match the dimension of the homology-modelled helicase domain ( Fig. 8a ). As a result, the assembly of the MHF–FANCM complex on branched DNA is expected to minimize unproductive association of FANCM with duplex DNA away from the junction and to enhance the efficiency of DNA branch migration by orienting the FANCM active site in the optimal geometry. Considering MHF’s biochemical role in stimulating the translocase activity of FANCM, such resemblance brings new possibility into MHF’s working mechanism. MHF might not only increase the FANCM-binding affinity to branched DNA substrates, but also confer some dynamic property to make the FANCM-MHF complex a fully functional translocase targeting branched DNA sites. 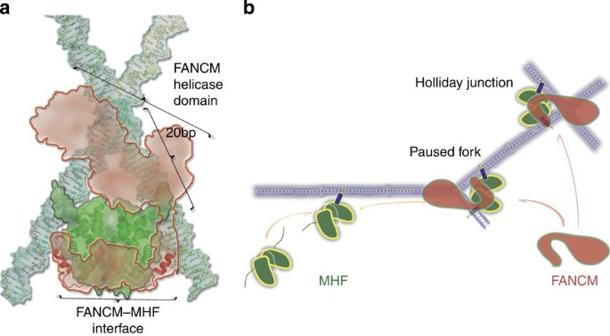Figure 8: Model for the function of MHF in the FA pathway of DNA damage repair. (a) The MHF–FANCM (661–800) structure (PDB ID: 4DRB) is overlaid onto the tetramer 1 in the MHF–DNA complex (FANCM in red, MHF in green and DNA in cyan). The ideal HJ DNA is shown as sticks. The homology-modelled helicase domain of FANCM is shown as semitransparent red contour. (b) Model depicting a role of MHF (green) in facilitating FANCM (red) to branched DNA (purple) in FA pathway of DNA repair. The arm regions are also displayed before (as blue wires) or after (or blue tailed tubes) DNA binding. Figure 8: Model for the function of MHF in the FA pathway of DNA damage repair. ( a ) The MHF–FANCM (661–800) structure (PDB ID: 4DRB) is overlaid onto the tetramer 1 in the MHF–DNA complex (FANCM in red, MHF in green and DNA in cyan). The ideal HJ DNA is shown as sticks. The homology-modelled helicase domain of FANCM is shown as semitransparent red contour. ( b ) Model depicting a role of MHF (green) in facilitating FANCM (red) to branched DNA (purple) in FA pathway of DNA repair. The arm regions are also displayed before (as blue wires) or after (or blue tailed tubes) DNA binding. Full size image The results presented herein provide a framework for understanding the mechanisms by which the conserved MHF complex engages various branched DNA structures and facilitates the FA pathway of genome maintenance and replication fork repair. Insight into the clinical impact of MHF is currently limited by the relatively rare occurrence of MHF mutations in patients. There are only 19 mutations, mostly missense substitutions, in MHF1 gene out of 7,741 unique samples in the Catalogue Of Somatic Mutations In Cancer (COSMIC) database ( http://www.sanger.ac.uk/genetics/CGP/cosmic/ ). Cancer linkage to MHF1 or MHF2 has not been identified. However, because of the important cellular functions of the MHF complex in FA pathway activation and DNA genome maintenance, it is possible that FA patients with mutations in MHF1 and MHF2 will be discovered in the future. Protein overexpression and purification The human MHF complex was expressed as described in ref. 13 . Briefly, Rosetta Escherichia coli BL21 (DE3) cells (Novagen) were transformed with a duet vector expressing both MHF1 (glutathione S -transferase (GST)-tagged) and MHF2 (6 × His-tagged) proteins. After cell lysis, the MHF complex was purified by a combination of Talon (Clontech), glutathione affinity (GE Healthcare), treatment with TEV (tobacco etch virus) protease to cleave off the GST tag on MHF1, hydroxyapatite (GE Healthcare), Mono Q (GE Healthcare) and Superdex S200 gel-filtration chromatography (GE Healthcare). The MHF mutants used in this study were generated using the QuickChange Site-Directed Mutagenesis kit (Stratagene), verified by DNA sequencing, expressed and purified using the same procedure. SeMet-containing MHF complex was expressed in B834 competent cells (Novagen) and grown in M9 minimal media (Sigma-Aldrich) containing SeMet (Sigma-Aldrich) and purified using the same procedure. MHF–DNA complex was obtained by mixing MHF tetramer with a DNA that enables the formation of duplex DNAs from the self-complementary sequence: 5′-ATCAATATCCACCGGTGGATATTGAT-3′ (Integrated DNA Technologies), in 2:1 molar ratio and further purified by gel-filtration chromatography on a Superdex 200 column buffered with 20 mM Tris, pH 8.0, 150 mM NaCl and 0.1 mM TCEP (tris-(2-carboxyethyl)phosphine. The FANCM-F fragment (661–800) was cloned in the pMAL-TEV (New England Biolabs) vector and expressed in Rosetta cells with an amino-terminal MBP (maltose-binding protein) tag. The protein was purified using amylose agarose (GE Healthcare), Mono Q and gel filtration in Superdex 200 column. The FANCM-F/MHF1–MHF2 complex was purified as follows. Cells expressing MBP-tagged FANCM-F and GST-tagged MHF1–MHF2 were mixed and an extract was prepared. Purification was achieved by glutathione and amylose affinity steps. TEV protease was mixed with protein eluted from the amylose resin (1:1,000 molar ratio) followed by an overnight incubation. The cleaved tags were removed by gel filtration in Superdex 200. Crystallization and structure determination The apo-MHF was crystallized using the macro-batch under oil method [26] . A mixture of protein and reservoir buffer was deposited under a layer of 2:1 paraffin (Fluka):silicon (Hampton Research) oil and allowed to equilibrate at room temperature. Crystals were obtained in crystallization buffers containing (a) 0.1 M sodium phosphate, pH 6.5, with 12% PEG8000, (b) 0.1 M HEPES, pH 7.0, with 20% PEG8000 and (c) 0.1 M magnesium chloride with 0.1 M HEPES, pH 7, and 15% PEG4000. The SeMet-containing MHF complex was crystallized under the same conditions. Crystals were frozen using 30% glycerol as a cryoprotectant. Diffraction data were collected at the Advanced Photon Source beamline 24-ID and the National Synchrotron Light Source beamline X29A. Data were processed and scaled using HKL2000 (ref. 27 ; Table 1 ). The structure was solved by a combination of SeMet single-wavelength anomalous dispersion and multiwavelength anomalous dispersion phasing at 2.1 Å resolution using Shelx [28] and Solve [29] . A twofold NCS averaging using DM [30] significantly improved the electron density map, which allowed Buccanneer [31] for automatic model building of 308 out of 438 total ASU residues. The model was subsequently refined using Phenix [32] and manually rebuilt in Coot [33] to a final R / R free of 0.230/0.262. The structures in the other two crystal forms were solved by molecular replacement (MR) using the model obtained for the SeMet data and refined to R / R free of 0.223/0.264 (MHF-apo1) and 0.231/0.252 (MHF-apo2), respectively. Data and refinement statistics are summarized in Table 1 . MHF–DNA crystals were grown in 0.5–0.7 M ammonium phosphate at room temperature using the macro-batch under oil method and then frozen in liquid nitrogen with 15% ethylene glycol added as a cryoprotectant. Diffraction data were collected at 100 K on beamline 24-IDC at the Advanced Photon Source. Data were processed using HKL2000 (MHF–DNA1 in Table 1 ) to 7.2 Å ( I / σ ~1, CC 1/2 ~0.14 by the Pearson’s correlation coefficient method [34] ) in space group P321. MR was performed in PHASER [30] , [35] using the MHF heterodimer as a search model. This gave an initial solution of three heterodimers ( Supplementary Fig. S2a ). Further, MR using a 13-bp ideal B-DNA model (generated by Coot with the sequence 5′-AAAAAAAAAAAAA-3′ in one strand and the complementary sequence in the other strand) yielded two solutions in a slightly misaligned head-to-tail geometry ( Supplementary Fig. S2b,c ). Subsequent refinement and density modification revealed a continuous double helical density, accommodating a 26-bp ideal B-DNA, at a position different from that of the initial 13 bp DNA model, confirming the electron density for the DNA is not model biased ( Supplementary Fig. S2c,d ). Further refinement and additional real-space MR search in the electron density located the last two MHF heterodimers in the crystal. Refinement was carried out using Phenix [32] and Refmac [36] using local restraints from a reference structure of apo-MHF [37] , jelly-body [18] and NCS [18] restraints, yielding a refined model with R / R free of 32.3/34.4% and good stereochemical geometry. A second, related crystal form of the MHF–DNA complex (MHF–DNA2) was obtained, which diffracted to 6.5 Å resolution ( I / σ ~0.5, CC 1/2 ~0.16 by the Pearson’s correlation coefficient method [34] ). The two crystals have very similar cell dimensions in a and b directions, but the cell constant in the c direction is doubled in MHF–DNA2. Inspection of the native Patterson map revealed a strong NCS translational peak of ~80% of the origin peak height at the fractional coordinates of (0, 0, 0.5). This is consistent with that the unit cell of MHF–DNA2 consists of two translationally related layers of molecules along the c axis. The molecules in each layer have virtually identical structures and packing environment as those in MHF–DNA1. The solution obtained in MHF–DNA1 was used as a search model to solve the structure of MHF–DNA2, which is subsequently refined to R / R free of 30.7/37.9%. A thorough inspection of the diffraction data revealed that both MHF–DNA complex crystals are twinned, with twinning fractions close to 0.5 ( Table 1 ) in the P3 space group, resulting in an apparent space group of P321. Interestingly, the conventional twinning tests, such as Wilson ratios and cumulative intensity distribution, did not detect twinning. This is presumably due to the high degree of NCS, especially the translational NCS in MHF–DNA2, which may alter the apparent intensity distribution. Nonetheless, the L test [38] and the maximum likelihood method implemented in Phenix Xtriage [32] clearly revealed twinning with the twining operator ‘ k , h , - l ’ ( Supplementary Fig. S8 ). Diffraction data for both MHF–DNA1 and MHF–DNA2 were reprocessed in the P3 space group. Care was taken to maintain a consistent and independent set of R free flags, with those from the P321 data kept and expanded based on the twinning operator using Phenix.reflection_tools [32] . The amplitude-based twin refinement in Refmac5 (ref. 18 ) resulted in a substantial decrease of R free factors of ~6% in both MHF–DNA crystal forms ( R / R free : 26.8/28.8% for MHF–DNA1 and 28.3/31.3% for MHF–DNA2). The slightly higher R factors of the MHF–DNA2 structure are probably due to the strong translational NCS in the crystal, as pseudotranslation is known to introduce artificially high R factors due to intensity modulations [39] , [40] . The B -factors of the refined structures are consistent with the Wilson B -factors calculated from the diffraction data ( Table 1 , Supplementary Table S2 and Supplementary Fig. S1b,c ), although Wilson statistics at low resolution are not accurate. The B -factors for the DNA and the protein components are similar, indicating similar ordering of these components in the crystals. More importantly, the twin refinement significantly improved the resulting electron density maps, exemplified by the appearance of unbiased difference electron density for the MHF1 C-terminal region without any model information ( Fig. 1b and Supplementary Fig. S2g ), which only appeared after successful twin refinement. Radiolabelled DNA substrate preparation Radiolabelled ds, fork, HJ and MRF substrates were prepared from synthetic oligos ( Supplementary Table S1 ). The DNA hybridization reactions were conducted by heating equimolar amounts of the indicated oligonucleotide mixture at 95 °C for 10 min in buffer H (50 mM Tris-HCl, pH 7.5, 10 mM MgCl 2 , 100 mM NaCl) followed by slow cooling to room temperature. DNA substrates were separated from un-annealed oligonucleotides in 10% non-denaturing polyacrylamide gels run in TAE buffer (40 mM Tris acetate, pH 7.4, 0.5 mM EDTA) and were recovered from the gel by electroelution in dialysis tubing in TAE buffer. DNA-binding assays WT and mutant-MHF complexes were incubated with various radiolabelled DNA substrates (dsDNA, MRF and HJ). The reaction mixtures were analysed by mixing protein with various concentration of DNA substrates. The concentration of MHF complex is calculated as molar concentration of the tetramer. Reactions were conducted in triplicates to obtain the mean and the s.d. values. For the DNA-binding competition assays, MHF or the FANCM-F/MHF complex was incubated with a mixture of ds-, forked and HJ DNAs at 30 nM molar concentration each in buffer (25 mM Tris, pH 7.5, 1 mM dithiothreitol, 100 μg ml −1 BSA) containing 150 mM KCl for 10 min at 37 °C. After addition of 5 μl loading buffer (50% glycerol, 20 mM Tris-HCl, pH 7.4, 2 mM EDTA, 0.05% orange G), the reaction mixtures were resolved in 6.5% native polyacrylamide gel in TBE buffer (45 mM Tris-borate, 1 mM EDTA, pH 8.0) at 4 °C. Gels were dried onto Whatman DE81 paper (Whatman International Limited) and then analysed in a Personal Molecular Imager FX PhosphorImager (Bio-Rad). Reactions were conducted in triplicates to obtain the mean and the s.d. values. Cold DNA competition assays For competition, the MHF complex (100 nM) was preincubated with 30 nM radiolabelled dsDNA substrate for 5 min at 37 °C. Subsequently, the indicated concentration of either unlabelled dsDNA or HJ DNA was added, followed by a 5-min incubation at 37 °C. The reaction mixtures were resolved and analysed as above. Reactions were conducted in triplicates to obtain the mean and the s.d. values. DNA branch migration assay The reactions (10 μl) for branch migration assays with MRF contained 10 nM protein with 5 nM DNA substrate in the presence of ATP. Reactions were carried out at 37 °C for the indicated periods. The resulting mixture were deproteinized for 20 min at 37 °C with 2 mg ml −1 Proteinase K and 0.4% SDS, and resolved by native PAGE through 8% polyacrylamide gels in TBE. Assays were conducted in triplicates to obtain the mean and the s.d. values. MHF and FANCM-F pull-down assay Ten micrograms of WT MHF or MHF mutant (K73A/R74A, K12A/H20A/K27A/K29A, K73A/K94A/K99A/R110A, K44A/R64A or R18A/R11A/R17A) was incubated with the same molar ratio of MBP-His-FANCM-F (FANCM fragment 661–800) and incubated in 30 μl of buffer (25 mM Tris-HCl at pH 7.5, 0.01% NP-40, 50 mM KCl, 1 mM dithiothreitol) for 1 h at 4 °C. Amylose agarose resin (10 μl; New England Biolabs) was added, followed by gentle mixing for 30 min at 4 °C. After washing the beads twice with 200 μl of buffer, bound proteins were eluted with 30 μl of 2% SDS. Fifteen per cent of the supernatant and elution fractions, and 2% of total wash fraction were analysed by 15% SDS–PAGE followed by Coomassie blue staining. Control experiments were conducted to show that the MHF mutants were not retained on the Amylose resin without the inclusion of the MBP-tagged FANCM-F. Homology modelling of the FANCM helicase domain A crystal structure (PDB ID: 1WP9) is available for Pyrococcus furiosus Hef [25] , the FANCM orthologue. Hef has 764 amino acid residues and 30/70% sequence identity/similarity to the corresponding helicase and C-terminal regions of FANCM. Because of the high sequence similarity, we were able to generate a homology model of the FANCM helicase domain based on the Hef crystal structure [25] using the automated modelling server I-TASSER [41] , which has consistently ranked as the top performer in the CASP (Critical Assessment of Techniques for Protein Structure Prediction) modelling contests. Tethered particle flow stretching WT or mutant-MHF was diluted to 10 μM in PBS with 1 mg ml −1 casein and 0.1% TWEEN, and injected into a flow cell with a depth of 0.5 mm and a width of 5 mm. Measurements were taken at the centre of the flow cell. To stretch the DNA, beads were tracked under a constant flow force of ~0.5 pN generated using a syringe pump (OEM syringe pump, Harvard Apparatus). The flow force was calibrated by measuring the mean displacement of the bead at various flow rates and then fitting to an experimentally calibrated worm-like chain model that relates the extension of the DNA-tethered beads with the measured force exerted by optical tweezers [42] . To obtain the flow force of ~0.5 pN, we first calculated the extension of the tethered bead predicted from the worm-like chain model [42] and subsequently tuned the flow rate to match the experimental extension ( Supplementary Fig. S4a ) to the theoretical prediction ( Supplementary Fig. S4b ). Detailed information regarding instrumental setup and calibration is in Supplementary Methods . The flow rate equivalent to ~0.5 pN force is 64 μl min −1 in our experimental setup, which was used for all TPFS assays on both WT MHF and MHF mutants. The measurements were repeated for a minimum of ten tethers in each case. As the measured total extension includes both the length of the DNA and the size/radius of the tethered bead, the apparent initial extensions can vary up to 20% from bead to bead due to the intrinsic variations in bead size. In addition, the difference in bead size results in a fluctuation in flow force from bead to bead. Despite the variations, the same length reduction (corresponding to ~1,400-bp long) from initial extension has been observed consistently on the addition of all MHF capable of DNA binding, but not for the DNA-binding-impaired MHF mutant, suggesting the same MHF-induced DNA condensation phenomenon. Initially, when few MHF molecules are bound, they are potentially in the single-side binding mode and there is little condensation occurring right away. This is probably because the DNA-bending, double-side binding energy is not enough to overcome the energy required for DNA bending under the experimental flow force. When enough MHF proteins bind, the collective binding energy overcomes the energy to bend the DNA and the DNA begins to condense. The initial bending will then bring duplex regions of the DNA close together, creating a geometry that facilitates the binding of the next MHF molecules. This continues until an equilibrium is reached in the experimental condition and condensation stops. This type of condensation has been observed with other DNA-binding proteins such as histone H1 (ref. 43 ). Antibodies and drug-sensitivity tests Anti-Flag (1:500), -MHF1 (1:1,000), -MHF2 (1:500), -FANCM (1:2,000), -FAAP24 (1:3,000) and -FANCD2 (1:4,000) antibodies were prepared and drug-sensitivity assays were performed. Two hundred HeLa cells transduced with lentiviruses carrying either control shRNA or shMHF1-UTR were seeded per 10-cm dish containing the indicated concentration of MMC or camptothecin (in Fig. 6c ). After 10 days, cells were fixed, stained and visible colonies were counted. Assays were conducted in triplicates to obtain the mean and the s.d. values. Co-immunoprecipitation of FANCM and MHF HeLa cells were transduced with lentiviruses carrying shMHF1-UTR (5′-GATAATGTGTACTGCGTTA-3′). The cells were subsequently transduced with retroviruses carrying empty vector (pMIEG3), Flag-WT-MHF1 or Flag-MHF1 mutant (K73A/K94A/K99A/R110A), and treated with 100 ng ml −1 MMC for 16 h. Cell lysate was prepared and treated with anti-FLAG resin (Sigma-Aldrich). Immunoprecipitated protein complexes were analysed by immunoblotting with the corresponding antibodies (anti-FLAG, -MHF2, -FAAP24 and -FANCM). Chromatin localization assay HeLa cells were transduced with lentiviruses carrying either control shRNA (SCB: 5′-CCTAAGGTTAAGTCGCCCTCG-3′) or shMHF1-UTR (5′-GATAATGTGTACTGCGTTA-3′). Next, Hela-MHF1-UTR cells were transduced with retroviruses carrying either an empty vector, shRNA-resistant WT-MHF1 complementary DNA or mutant MHF (K73A/K94A/K99A/R110A). Cells were treated with 100 ng ml −1 MMC for 16 h, followed by cellular fractionation into total lysate and chromatin fraction. Cell-equivalent volumes from total cell lysate and chromatin fraction were separated by SDS–PAGE and immunoblotted with antibodies. Uncropped images of the western blottings can be found in Supplementary Fig. S9a . FANCD2 activation assay HeLa cells were transduced with lentiviruses carrying either control shRNA or shMHF1-UTR. Subsequently, cells were transduced with retroviruses carrying empty vector (pMIEG3), shRNA-resistant WT-MHF1 cDNA or mutant-MHF (K73A/K94A/K99A/R110A). Enhanced green fluorescent protein-positive cells were sorted by FACS analysis. Cells were treated with 100 ng ml −1 MMC for 16 h, lysed and immunoblotted with anti-FANCD2 antibody(1:4,000). Uncropped images of the western blottings can be found in Supplementary Fig. S9b . Data deposition: The atomic coordinates and structure factors for the apo-MHF1–MHF2 and MHF1–MHF2–DNA structure have been deposited in the Protein Data Bank with accession codes: 4NE6 (MHF-Se), 4NE5 (MHF-apo1), 4NE3 (MHF-apo2), 4NE1 (MHF–DNA2) and 4NDY (MHF–DNA1). How to cite this article: Zhao, Q. et al. The MHF complex senses branched DNA by binding a pair of crossover DNA duplexes. Nat. Commun. 5:2987 doi: 10.1038/ncomms3987 (2014).